Caesium accumulation in yeast and plants is selectively repressed by loss of the SNARE Sec22p/SEC22 The non-essential cation caesium (Cs + ) is assimilated by all organisms. Thus, anthropogenically released radiocaesium is of concern to agriculture. Cs + accumulates owing to its chemical similarity to the potassium ion (K + ). The apparent lack of a Cs + -specific uptake mechanism has obstructed attempts to manipulate Cs + accumulation without causing pleiotropic effects. Here we show that the SNARE protein Sec22p/SEC22 specifically impacts Cs + accumulation in yeast and in plants. Loss of Saccharomyces cerevisiae Sec22p does not affect K + homeostasis, yet halves Cs + concentration compared with the wild type. Mathematical modelling of the uptake time course predicts a compromised vacuolar Cs + deposition in sec22Δ . Biochemical fractionation confirms this and indicates a new feature of Sec22p in enhancing non-selective cation deposition. A developmentally controlled loss-of-function mutant of the orthologous Arabidopsis thaliana SEC22 phenocopies the reduced Cs + uptake without affecting plant growth. This finding provides a new strategy to reduce radiocaesium entry into the food chain. Cs + is considered to be non-essential for organisms. As it is the rarest alkali cation that does not accumulate in soil, no detrimental effects are ascribed to Cs + in natural conditions. However, it has acquired enormous ecological importance owing to the anthropogenic release of its persisting radioisotope 137 Cs ( T ½ =30.1 years), in particular by catastrophic events like the nuclear meltdown and explosions of the Chernobyl or Fukushima nuclear power plants [1] , [2] . Among the alkali metal cations, K + , Rb + and Cs + have comparable physico-chemical characteristics owing to similar radii of their hydrated ions [3] . Therefore, Cs + and Rb + uptake is mediated by potassium transport systems and Cs + radioisotopes easily enter the food chain via plants [4] , [5] . Agriculture in contaminated areas needs to be restricted or remediation strategies have to be developed [6] . Bioremediation could be based on plants accumulating higher amounts of Cs + . Conversely, it has been suggested to reduce Cs + input into the food chain by developing ‘safer crops’, which discriminate against Cs + (ref. 7 ). To this end, Cs + uptake has been intensely studied in plants. Uptake and transport across root plasma membranes are considered to be the key aspect and thereby a promising target for manipulating Cs + uptake [5] . High-affinity Cs + uptake has been attributed to HAK/KUP-type K + transporters [5] . Low-affinity uptake, although less relevant for ecological scenarios, can be mediated through CNGC-type channels [5] . Mutual interference of Cs + with K + or Rb + accumulation has further substantiated it as a substrate for K + uptake proteins in plants and other organisms [5] , [6] , [8] , [9] . However, Cs + exhibits toxicity already at a rather low concentration with respect to the high intracellular K + concentration, whereas Rb + can even replace K + in a potassium-depleted scenario [10] . Previous studies have shown that Cs + may either inhibit or compete with K + -dependent processes, and that K + and Cs + concentrations are not strictly correlated [9] , [11] , [12] . Therefore, alternative transport processes may enable a discrimination between these closely related cations. Nevertheless, attempts to specifically manipulate Cs + accumulation in plants have failed owing to interference with K + homeostasis leading to detrimental, pleiotropic effects [5] . A discriminative uptake mechanism for a non-essential and rare cation would also be surprising from an evolutionary point of view, as toxic concentrations are not reached in nature. Therefore, a biotechnological approach based on mutagenesis should target crucial root uptake and/or export proteins to achieve an improved K + /Cs + specificity and selectivity [5] . In addition, recent analyses of the natural genetic variation of Cs + accumulation have revealed several quantitative trait loci in A. thaliana accessions, which might be helpful for determining additional, possibly multigenic, factors in Cs + homeostasis [13] , [14] . The yeast S. cerevisiae provides a unicellular and simple test system to study Cs + uptake, as it has been shown to utilize cation transporters and channels similar to plant cells [8] . We have recently employed an unbiased approach to identify candidate genes compromising Cs + accumulation by screening a yeast-knockout collection [15] . Vacuolar maintenance and vesicle transport are the highest enriched categories among the identified genes. Here, we characterize the mutant sec22Δ in more detail. It specifically reduces the accumulation of Cs + , as the homeostasis of K + and other cations is not affected. Sec22p is a well-described non-essential yeast SNARE involved in the anterograde and retrograde vesicle membrane fusion at the endoplasmic reticulum (ER)–Golgi interface and in autophagy [16] , [17] . Modelling of Cs + uptake time course points to vacuolar sequestration as a crucial factor, which is compromised in the sec22Δ mutant and thereby indicating a novel feature of Sec22p function in yeast. Although the A. thaliana ortholog SEC22 had been shown to be required for gametophyte development [18] , we succeeded in identifying a sec22 mutant allele, which only affected vegetative tissues and phenocopied the specific repression of Cs + accumulation. The plant gene partially complements the yeast mutant indicating a conserved mechanism. We therefore propose that this novel Sec22p/SEC22-dependent function will provide a new route to generate ‘safer crops’. Cs + accumulation is specifically reduced in sec22Δ Previously, we have screened a loss-of-function mutant collection of S. cerevisiae for altered uptake of Cs + (ref. 15 ). The categories ‘vacuolar function’ and ‘vesicle-mediated transport’ are enriched among the mutants that show reduced Cs + concentration. Three of these mutants, vps35Δ , aps3Δ and apl4Δ , do not significantly affect the K + content [15] . However, we have found that all of them exhibited pleiotropic effects ( Supplementary Fig. S1 ). Therefore, we have considered further candidates with reduced Cs + uptake searching for both a non-pleiotropic behaviour and the existence of homologous genes, which would allow a potential functional analysis in plants. Among them, sec22Δ exhibits wild-type-like growth and viability ( Supplementary Fig. S1 ). Furthermore, Sec22p-like proteins are conserved in higher organisms including plants ( Supplementary Fig. S2a ). 134 Cs tracer studies confirm that sec22Δ accumulates less than half of Cs + as compared with the wild type ( Fig. 1a ). In contrast, the potassium analogue Rb + accumulates to similar concentrations. The concentrations of essential cations (K + , Na + , Ca 2+ and Mg 2+ ) remain unaltered. Complementation with the wild-type gene suppresses this Cs + -discriminative phenotype ( Fig. 1a ). Thus, the loss of SEC22p (YLR268Wp) does not disturb growth and viability, but specifically reduces Cs + concentration without affecting the content in K + and other essential cations. In contrast to the lower Cs + accumulation, sec22Δ displays a slightly increased sensitivity towards Cs + ( Fig. 1d ). 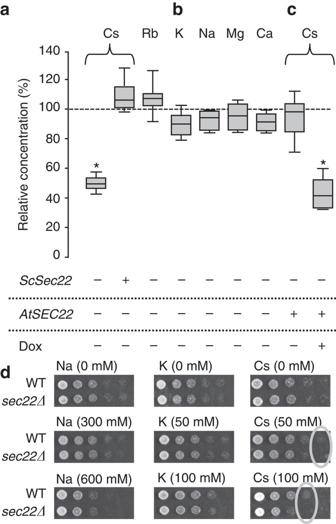Figure 1: Cs+-specific repression of cation accumulation in the yeast mutantsec22Δ. (a) Cs+and Rb+uptake by thesec22Δmutant and a complemented strain (ScSec22+).134Cs and86Rb cation concentrations were determined from 107cells after 18 h in YPD containing 50 μM 5-FU and 50 μM CsCl. The wild-type reference strain BY4741 contained 2.1±0.1 mM Cs+or 2.3±0.6 mM Rb+. (b) K+, Na+, Ca2+and Mg2+concentrations were retained in thesec22Δmutant under these conditions. Wild-type concentrations were 164±9.7 mM K+, 2.7±0.1 mM Na+, 31.4±0.3 mM Mg2+and 1.2±0.1 mM Ca2+. (c) Complementation ofsec22ΔCs+uptake deficiency byA. thaliana SEC22expressed under the control of a doxycycline-repressible promoter. Presence or absence ofS. cerevisiae Sec22orA. thaliana SEC22expression, as well as addition of doxycycline, is indicated by +/−. (a–c) Box plots are displayed (n=10); quartiles define the box limits and antennas denote maximum and minimum values; asterisks indicate significant differences from wild type (P≤0.001,t-test). (d) Toxicity test of wild type andsec22Δin dilution series (1/1, 1/5, 1/25, 1/125 and 1/625) at different concentrations of alkali cations in YPD agar pH 6. Grey circles indicate dilutions at whichsec22Δshows higher sensitivity than wild type. Colony sizes, 7–8 mm. Figure 1: Cs + -specific repression of cation accumulation in the yeast mutant sec22Δ . ( a ) Cs + and Rb + uptake by the sec22Δ mutant and a complemented strain ( ScSec22 +). 134 Cs and 86 Rb cation concentrations were determined from 10 7 cells after 18 h in YPD containing 50 μM 5-FU and 50 μM CsCl. The wild-type reference strain BY4741 contained 2.1±0.1 mM Cs + or 2.3±0.6 mM Rb + . ( b ) K + , Na + , Ca 2+ and Mg 2+ concentrations were retained in the sec22Δ mutant under these conditions. Wild-type concentrations were 164±9.7 mM K + , 2.7±0.1 mM Na + , 31.4±0.3 mM Mg 2+ and 1.2±0.1 mM Ca 2+ . ( c ) Complementation of sec22Δ Cs + uptake deficiency by A. thaliana SEC22 expressed under the control of a doxycycline-repressible promoter. Presence or absence of S. cerevisiae Sec22 or A. thaliana SEC22 expression, as well as addition of doxycycline, is indicated by +/−. ( a – c ) Box plots are displayed ( n =10); quartiles define the box limits and antennas denote maximum and minimum values; asterisks indicate significant differences from wild type ( P ≤0.001, t -test). ( d ) Toxicity test of wild type and sec22Δ in dilution series (1/1, 1/5, 1/25, 1/125 and 1/625) at different concentrations of alkali cations in YPD agar pH 6. Grey circles indicate dilutions at which sec22Δ shows higher sensitivity than wild type. Colony sizes, 7–8 mm. Full size image Interestingly, wild-type yeast cells accumulate Cs + following a two-phase kinetics distinct from the hyperbolic uptake described for K + / Rb + (ref. 19 ). The uptake of Cs + comprises an initial step reaching about 0.35 mM at 2–3 h and a second step reaching a plateau at 2.2 mM cellular Cs + after >16 h ( Fig. 2a ). The time course of sec22Δ Cs + accumulation is highly similar to that of the wild type during the initial phase of about 2.5 h ( Fig. 2a–c ). However, further uptake is repressed and a lower steady-state concentration of ~1.1 mM Cs + is reached ( Fig. 2b ). 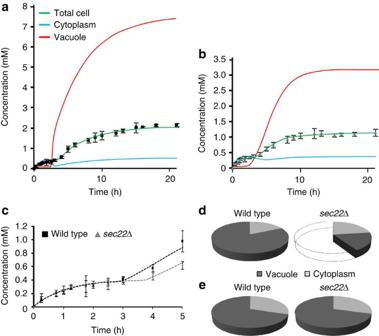Figure 2: Time course of Cs+accumulation in wild-type andsec22Δ-mutant yeast. Whole-cell Cs+concentrations were recorded at the indicated times after the addition of 50 μM CsCl. (a) Wild-type time course. (b)sec22Δtime course. Note the different scale of the concentration in (a) and (b). Continuous lines represent the fitting of the experimental data by the mathematical modelling and the predictions for the compartmentalization: the total intracellular (green), the cytoplasmic (blue) and the vacuolar (red) concentrations are depicted (Supplementary Methods). Steady-state Cs+concentrations were predicted at 2.1 mM (wild type) or 1.1 mM (sec22Δ) in whole cells, at 0.40 mM (wild type) or 0.39 mM (sec22Δ) in the cytoplasm, and at 7.1 mM (wild type) or 3.2 mM (sec22Δ) in vacuoles. (c) Overlay of the initial time courses of wild type andsec22Δ. (a–c) Data are presented as means±s.d. (n=10). (d) Scheme of relative Cs+compartmentalization in wild type andsec22Δ. Total Cs+accumulation and vacuolar Cs+compartmentalization were determined from whole cells after 18 h incubation in YPD supplemented with 50 μM radiolabelled Cs+. One complete pie represents 75 amol Cs+per cell (complete uptake of wild-type cells). Total amount and vacuolar partitioning of Cs+had been measured and were related to equal activity of the vacuolar marker α-mannosidase, resulting in a vacuolar Cs+deposition of ~82% (wild type) and 55% (sec22Δ), respectively;n=3 independent vacuole isolations. (e) Scheme of relative Rb+compartmentation measured in parallel to Cs+distribution. The complete pie represents 81 amol per cell (wild type) and 87 amol per cell (sec22Δ). Rb+deposition to the vacuole (70%) was identical for wild type andsec22Δ;n=3. Figure 2: Time course of Cs + accumulation in wild-type and sec22Δ -mutant yeast. Whole-cell Cs + concentrations were recorded at the indicated times after the addition of 50 μM CsCl. ( a ) Wild-type time course. ( b ) sec22Δ time course. Note the different scale of the concentration in ( a ) and ( b ). Continuous lines represent the fitting of the experimental data by the mathematical modelling and the predictions for the compartmentalization: the total intracellular (green), the cytoplasmic (blue) and the vacuolar (red) concentrations are depicted ( Supplementary Methods ). Steady-state Cs + concentrations were predicted at 2.1 mM (wild type) or 1.1 mM ( sec22Δ ) in whole cells, at 0.40 mM (wild type) or 0.39 mM ( sec22Δ ) in the cytoplasm, and at 7.1 mM (wild type) or 3.2 mM ( sec22Δ ) in vacuoles. ( c ) Overlay of the initial time courses of wild type and sec22Δ . ( a – c ) Data are presented as means±s.d. ( n =10). ( d ) Scheme of relative Cs + compartmentalization in wild type and sec22Δ . Total Cs + accumulation and vacuolar Cs + compartmentalization were determined from whole cells after 18 h incubation in YPD supplemented with 50 μM radiolabelled Cs + . One complete pie represents 75 amol Cs + per cell (complete uptake of wild-type cells). Total amount and vacuolar partitioning of Cs + had been measured and were related to equal activity of the vacuolar marker α-mannosidase, resulting in a vacuolar Cs + deposition of ~82% (wild type) and 55% ( sec22Δ ), respectively; n =3 independent vacuole isolations. ( e ) Scheme of relative Rb + compartmentation measured in parallel to Cs + distribution. The complete pie represents 81 amol per cell (wild type) and 87 amol per cell ( sec22Δ ). Rb + deposition to the vacuole (70%) was identical for wild type and sec22Δ ; n =3. Full size image Modelling proposes impaired vacuolar Cs + deposition in sec22Δ To gain further understanding of the Cs + uptake and how sec22Δ leads to the lower Cs + accumulation, we have developed a mathematical model to describe the time course of wild-type and mutant high-affinity Cs + uptake. Cs + has been shown to be deposited into the vacuole of yeast cells [8] . Therefore, a minimal model comprises three compartments with defined volumes, the extracellular medium ( V 1 ), the cytoplasm ( V 2 ) and the vacuole ( V 3 ). Cellular and vacuolar volumes have been microscopically determined to be ~35 fl and 9 fl, respectively, and thus the cytoplasmic volume V 2 should be 26 fl. The respective volumes do not significantly differ between wild type and mutant ( Fig. 3a ). Two inward and outward fluxes into and from the cytoplasm (with rate constants k 1 and k 2 , respectively), as well as further possible sequestration into and from the vacuole (with rate constants k 3 and k 4 , respectively), with a linear dependence on Cs + concentrations are assumed ( Supplementary Fig. S3 ). In addition, the model allows for a potential delay of the vacuolar deposition by introducing a time-dependent upregulation s(t) of the flux towards the internal compartment. A deterministic model consisting of ordinary differential equations for the time dependence of the cellular Cs + concentration tot (t) has been developed. This model allows for fitting the experimental data, as well as for predicting cytoplasmic x(t) and vacuolar y(t) Cs + concentrations as expressed by the following equations ( Fig. 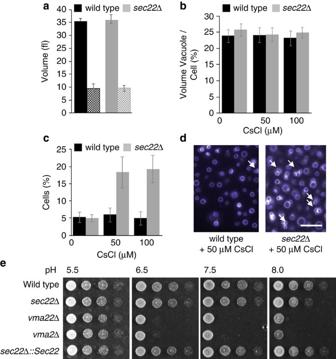Figure 3: Characterization ofsec22Δvacuoles. Morphology of vacuoles and pH sensitivity were analysed insec22Δand wild type. (a) Cellular (filled bars) and vacuolar (squares) volumes. In case of several vacuolar lobes stained per cell, the volumes of the lobes were added. Cell volumes are 35.2±1.2 fl (wild type) and 35.8±1.7 fl (sec22Δ); and vacuolar volumes are 8.8±0.9 fl and 9.0±1.2 fl. FM4-64 staining was used to label vacuoles in living yeast cells. Fifty cells from three independent cultivations were evaluated. Data are presented as means±s.d. (b) Percent ratio of vacuolar to cellular volumes at different external Cs+concentrations (n=30 cells). Data are presented as means±s.d. (c) Cells with fragmented vacuoles at three different concentrations of external CsCl, as well as at 100 mM external KCl. Cells showing two to five smaller sized lobes were defined as fragmented in contrast to a regular anatomy with a single, large vacuole. Data are presented as means±s.d. (n=3 with 100 cells in each independent replicate). All analyses in (a,b,c) were performed in YPD-rich medium after addition of cytostatic 5-FU. Both the absolute and relative vacuolar volumes, as well as vacuolar morphology, were similar in wild type andsec22Δ.However, at experimental conditions (50 μM Cs+)sec22Δhas a significantly higher percentage of fragmented vacuoles (18.3±4.5%) than wild type (6.0±2.1%) (P≤0.01), which has also been confirmed at 100 μM Cs+. (d) Wild-type and mutant cells grown in the presence of 50 μM CsCl. Normal and fragmented (white arrows) vacuoles are visualized by FM4-64 fluorescence. Scale bar: 10 μm. (e) pH sensitivity of yeast strains. Wild type,sec22Δ,vma22Δ,vma2Δandsec22Δ::Sec22(sec22Δcomplemented with wild-typeSec22) were tested on YPD plates buffered at different pH (dilution series 1/1, 1/5, 1/25, 1/125 and 1/325). Colony sizes, 7–8 mm. 2a–c ; Supplementary Methods ): Figure 3: Characterization of sec22Δ vacuoles. Morphology of vacuoles and pH sensitivity were analysed in sec22Δ and wild type. ( a ) Cellular (filled bars) and vacuolar (squares) volumes. In case of several vacuolar lobes stained per cell, the volumes of the lobes were added. Cell volumes are 35.2±1.2 fl (wild type) and 35.8±1.7 fl ( sec22Δ ); and vacuolar volumes are 8.8±0.9 fl and 9.0±1.2 fl. FM4-64 staining was used to label vacuoles in living yeast cells. Fifty cells from three independent cultivations were evaluated. Data are presented as means±s.d. ( b ) Percent ratio of vacuolar to cellular volumes at different external Cs + concentrations ( n =30 cells). Data are presented as means±s.d. ( c ) Cells with fragmented vacuoles at three different concentrations of external CsCl, as well as at 100 mM external KCl. Cells showing two to five smaller sized lobes were defined as fragmented in contrast to a regular anatomy with a single, large vacuole. Data are presented as means±s.d. ( n =3 with 100 cells in each independent replicate). All analyses in ( a,b,c ) were performed in YPD-rich medium after addition of cytostatic 5-FU. Both the absolute and relative vacuolar volumes, as well as vacuolar morphology, were similar in wild type and sec22Δ. However, at experimental conditions (50 μM Cs + ) sec22Δ has a significantly higher percentage of fragmented vacuoles (18.3±4.5%) than wild type (6.0±2.1%) ( P ≤0.01), which has also been confirmed at 100 μM Cs + . ( d ) Wild-type and mutant cells grown in the presence of 50 μM CsCl. Normal and fragmented (white arrows) vacuoles are visualized by FM4-64 fluorescence. Scale bar: 10 μm. ( e ) pH sensitivity of yeast strains. Wild type, sec22Δ , vma22Δ , vma2Δ and sec22Δ::Sec22 ( sec22Δ complemented with wild-type Sec22 ) were tested on YPD plates buffered at different pH (dilution series 1/1, 1/5, 1/25, 1/125 and 1/325). Colony sizes, 7–8 mm. Full size image with τ = k 3 /Γ=1− k 4 /Γ, Γ= k 3 + k 4 , =50 μM and the Hill function . For wild type, the model predicts a rapid increase of the cytoplasmic Cs + concentration with well-defined rate constants k 1 and k 2 , and a delayed sequestration to the vacuole with large, but less assessable, rate constants ( Supplementary Table S1 ; Supplementary Methods ). Fitting the wild-type experimental data, the model estimates Cs + concentrations of 0.4 mM in the cytoplasm and of 7.1 mM in the vacuole at the saturation of Cs + uptake ( Fig. 2a ). Fitting the sec22Δ mutant data results in an insignificantly altered rate constant k 1 ( P ≈1), an only slightly changed k 2 ( P =0.02) and again a delayed sequestration to the vacuole ( Supplementary Tables S1, S2 and S4 ). However, in contrast to the wild type, the model predicts a significantly compromised deposition of Cs + to sec22Δ vacuoles reaching only 3.2 mM (indicated by P ( τ )=1.15 × 10 −11 ) at a cytosolic Cs + concentration similar to wild type ( Fig. 2a ; Supplementary Table S1 ). Thus, the model indicates that the observed sec22Δ phenotype results from reduced vacuolar Cs + deposition. Reduced Cs + accumulation in sec22Δ vacuoles validates model To test the predictions of the mathematical model on vacuolar Cs + deposition, Cs + -laden vacuoles have been isolated from wild-type and mutant cells, and the sequestered portions of Cs + relative to whole-cell lysates have been measured. Wild-type and mutant cells contain similar amounts of the secretory system-independent vacuolar marker α-mannosidase in yeast [20] , which has been used to normalize the Cs + analyses ( Supplementary Fig. S4 ). The total Cs + taken up into wild-type cells (75 amol per cell at a concentration of 2.1 mM) is partitioned to the cytoplasm at a concentration of 0.78 mM and to the vacuole at 6.9 mM. Accordingly, ~82% of the total Cs + is deposited into the vacuole ( Fig. 2d ). This high recovery of Cs + also indicates that potential losses during the isolation procedure have been successfully avoided. The number is also in agreement with previous analyses of Cs + compartmentation [21] , but nevertheless may represent a lower limit of the vacuolar content. In contrast, sec22Δ (39 amol per cell; 1.1 mM) shows a cellular compartmentation of 0.66 mM Cs + in the cytoplasm and 2.4 mM in the vacuole. The potassium analogue Rb + is similarly partitioned to cytoplasm and vacuole of wild-type and mutant cells ( Fig. 2e ). Thus, the general reduction of Cs + accumulation by sec22Δ is owing to a specifically compromised partitioning to the vacuole, which contains only about one-third of the wild-type amount (22 amol per cell in comparison to 62 amol in wild type). This result is in good agreement with the predictions of the mathematical model ( Fig. 2a ). The reduction of Cs + uptake is not owing to a decrease in vacuolar volume or cell size, as both are not differentially influenced in wild-type and mutant cells after incubation in Cs + -containing YPD medium ( Fig. 3a ). In contrast, Jorgensen et al. [22] have reported an even slightly increased median cell size of sec22Δ . However, we have observed a higher frequency of cells harbouring several smaller vacuoles in the mutant, which is not evident in cells grown without Cs + ( Fig. 3c ). Thus, there is a Cs + -dependent morphological effect on sec22Δ vacuoles. The model also suggests that the reduced Cs + uptake of sec22Δ does not depend on differences at the plasma membrane ( Supplementary Table S1 ). We have addressed this issue by recording the loss of Cs + tracer from Cs + -laden cells at equilibrium conditions for 2 h after substituting the external tracer by unlabelled Cs + . The initial rate of efflux from wild-type and mutant cells at t =0 h was 0.62±0.11 mM h −1 and 0.52±0.09 mM h −1 , respectively. Thus, the efflux is not significantly altered in sec22Δ ( P =0.34; Supplementary Fig. S5 ). The magnitudes of the modelled efflux rates (wild type: 1.2 h −1 × 0.40 mM=0.48 mM h −1 ; sec22Δ : 1.9 h −1 × 0.39 mM=0.74 mM h −1 ) ( Fig. 2a ; Supplementary Table S1 ) are in agreement with these experimentally determined values. In summary, these results are in accordance with the prediction of similar Cs + fluxes at the plasma membrane in wild type and sec22Δ . Cs + uptake of cation transport mutants differs from sec22Δ To further explore and validate the results on the repressed Cs + accumulation and vacuolar sequestration in sec22Δ , additional mutants with known defects in cation import and export have been employed to analyse their impact on Cs + uptake. The time course of Cs + uptake has been recorded for trk1Δ , trk2Δ and trk1Δ trk2Δ , as well as for ena1-4Δ . The high-affinity transporter Trk1p and its homologue Trk2p are involved in potassium uptake at the plasma membrane; the Ena1-4 gene cluster encodes ATPases related to cation efflux [23] , [24] . In all cases except trk2Δ , the uptake time courses of these mutants primarily affecting the cation transport at the plasma membrane are considerably different from the respective wild types and, importantly, from sec22Δ ( Figs 2 and 4 ). Thus, these analyses support the divergent role of Sec22p in Cs + accumulation. 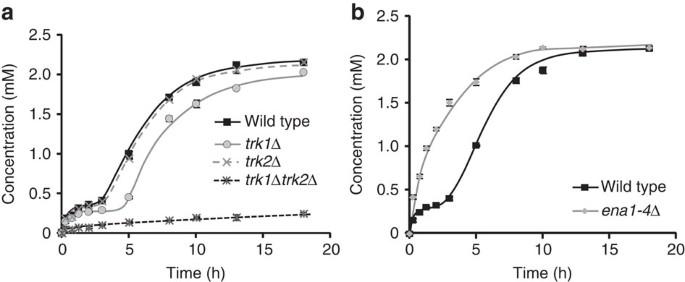Figure 4: Time course of Cs+accumulation in cation import- and export-impaired mutant yeast strains. The time course of whole-cell Cs+concentrations have been recorded at the indicated times after the addition of 50 μM CsCl to mutants affecting cation transport at the plasma membrane and their corresponding wild types. (a,b) Data are presented as means±s.d. (n=10). Continuous lines represent the fitting of the cellular Cs+concentrations by the mathematical model (Supplementary Methods). (a) Time course oftrk1Δ,trk2Δandtrk1Δtrk2Δand their corresponding wild type. (b) Time courses ofena1-4Δand its corresponding wild type. Figure 4: Time course of Cs + accumulation in cation import- and export-impaired mutant yeast strains. The time course of whole-cell Cs + concentrations have been recorded at the indicated times after the addition of 50 μM CsCl to mutants affecting cation transport at the plasma membrane and their corresponding wild types. ( a , b ) Data are presented as means±s.d. ( n =10). Continuous lines represent the fitting of the cellular Cs + concentrations by the mathematical model ( Supplementary Methods ). ( a ) Time course of trk1Δ , trk2Δ and trk1Δtrk2Δ and their corresponding wild type. ( b ) Time courses of ena1-4Δ and its corresponding wild type. Full size image The mutant trk1Δ leads to an attenuated increase in Cs + and a longer initial phase until further accumulation reaches almost wild-type level after 18 h, whereas the uptake trajectory of trk2Δ is almost indistinguishable from wild type ( Fig. 4a ). Thus, this data clearly demonstrate that (i) Trk1p is involved in Cs + uptake and (ii) Trk2p does apparently not contribute as long as Trk1p or other mechanisms are effective. However, the combined presence of Trk1p and Trk2p is required for efficient Cs + uptake, as within the time course analysed Cs + accumulation is drastically suppressed in trk1Δ trk2Δ ( Fig. 4a ). We have also fitted these uptake data using the mathematical model described above, yet employing the knowledge on the specific defects of trk1Δ and trk2Δ in cation influx by assuming an unchanged wild-type-like efflux at the plasma membrane. In all cases, the predicted Cs + sequestration to the vacuole is similar. The modelled influx rate constants k 1 are unaltered for trk2Δ , but slightly reduced for trk1Δ and strongly repressed for trk1Δ trk2Δ ( Supplementary Table S3 ). Interfering with plasma membrane cation efflux through the ena1-4Δ mutant leads to a strongly accelerated Cs + uptake and the apparent loss of the initial phase of the wild-type time course. However, a steady-state Cs + concentration similar to wild type is reached, although at an earlier time point ( Fig. 4b ). This experiment clearly supports a physiological role of Ena1-4p in Cs + efflux at the plasma membrane; its loss allows a more rapid Cs + accumulation. Fitting these data with the mathematical model, in this case assuming an intact, wild-type-like influx rate constant k 1 , predicts a reduced rate k 2 in accordance with the proposed biological function of Ena1-4p ( Supplementary Table S4 ). In addition, the limitation to wild-type-like steady-state Cs + concentration suggests that the ena1-4Δ mutation should also have other unknown consequences apart from an effect on the plasma membrane efflux. SEC22 in A. thaliana affects Cs + accumulation We employed the model plant A. thaliana to investigate whether the sec22Δ -dependent repression of Cs + uptake in a unicellular eukaryote would also be observed in a higher plant. SEC22 ( At1g11890 ) encodes a protein with 36% identity at the amino-acid level when compared with yeast Sec22p, sharing all functional domains ( Supplementary Fig. S2b ). It has been characterized as a SNARE involved in the anterograde vesicle traffic at the ER to Golgi interface [25] . In contrast to its S. cerevisiae ortholog, A. thaliana SEC22 is essential, as it is required for gametophyte development [18] . However, we have succeeded in recovering a fully viable and fertile, developmentally controlled loss-of-function mutant allele sec22-3 containing a T-DNA insertion in the 5′-UTR of At1g11890 (SALK_042819; Fig. 5a and Fig. 6 ). Reverse transcription PCR (RT–PCR) analyses reveal that this allele selectively lacks functional transcripts in vegetative tissue (root, stem and leaves), but retains expression in reproductive organs and young tissue probably due to a cryptic promoter activity of the T-DNA insert ( Fig. 5b ). The sec22-3 mutant has been examined for altered Cs + accumulation. It is reduced to about one half of wild-type concentration in rosette leaves and by about one-third in roots, while the Rb + , K + , Na + , Mg 2+ and Ca 2+ contents remain unaltered ( Fig. 7 ). Complementation with wild-type Arabidopsis SEC22 suppresses the phenotype. This demonstrates that the results obtained with yeast sec22Δ are phenocopied by the plant mutant suggesting a similar functional involvement in Cs + enrichment. To address this equivalence, Arabidopsis SEC22 has been cloned in a doxycycline-repressible expression vector ( Supplementary Methods ) and transiently expressed in the yeast mutant sec22Δ . Arabidopsis SEC22 is able to revert the low Cs + accumulation of sec22Δ reaching ~85% of the wild-type level. This reversion is abolished by suppressing the transgene expression with doxycycline ( Fig. 1c ). Thus, the plant SEC22 gene is able to functionally complement the yeast sec22Δ mutant. 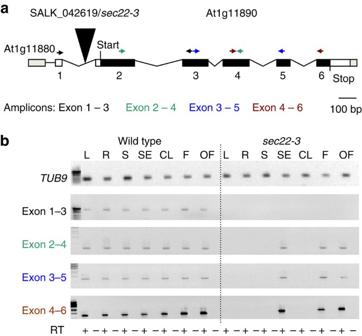Figure 5: Developmentally controlled loss ofSEC22transcription insec22-3. (a) The genomic structure ofAt1g11890is schematically shown including the position of the T-DNA insertion in thesec22-3allele (SALK_042619). Coloured arrows indicate forward and reverse primers used to amplify the marked exon combinations by RT–PCR. (b) RT–PCR-based analysis ofSEC22transcription in wild-type andsec22-3leaves (L), roots (R), stems (S), one-week-old seedlings (SE), cauline leaves (CL), flowers at stage 7–9 (F) and open flowers (OF, stage 14, with silique in early stage)60. Four differentSEC22exon combinations as defined in (a) were probed.A. thaliana TUB9transcription was used as a positive control; all combinations were tested +/− reverse transcriptase.pUC19cut byMspI (forTUB9andexon 1-3) or λ DNA cut byHindIII were used as size markers (at the left); amplicon sizes:TUB9, 184 bp; exon 1–3, 350 bp; exon 2–4, 410 bp; exon 3–5, 318 bp; and exon 4–6, 256 bp. Figure 5: Developmentally controlled loss of SEC22 transcription in sec22-3 . ( a ) The genomic structure of At1g11890 is schematically shown including the position of the T-DNA insertion in the sec22-3 allele (SALK_042619). Coloured arrows indicate forward and reverse primers used to amplify the marked exon combinations by RT–PCR. ( b ) RT–PCR-based analysis of SEC22 transcription in wild-type and sec22-3 leaves (L), roots (R), stems (S), one-week-old seedlings (SE), cauline leaves (CL), flowers at stage 7–9 (F) and open flowers (OF, stage 14, with silique in early stage) [60] . Four different SEC22 exon combinations as defined in ( a ) were probed. A. thaliana TUB9 transcription was used as a positive control; all combinations were tested +/− reverse transcriptase. pUC19 cut by Msp I (for TUB9 and exon 1-3 ) or λ DNA cut by Hin dIII were used as size markers (at the left); amplicon sizes: TUB9 , 184 bp; exon 1–3, 350 bp; exon 2–4, 410 bp; exon 3–5, 318 bp; and exon 4–6, 256 bp. 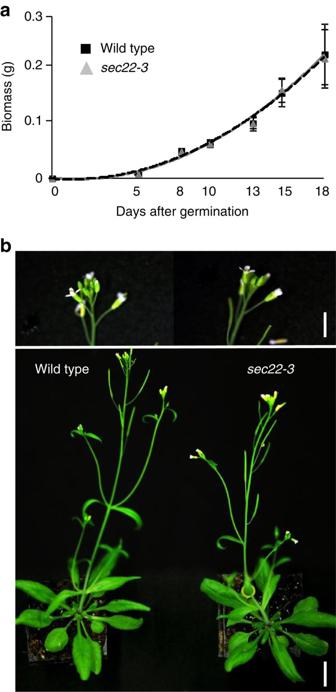Figure 6: Growth ofA. thalianawild type andsec22-3. (a) Plant development was quantified by measuring biomass (fresh weight) of aerial parts at the indicated time points (n≥15). Fresh weight to dry weight ratio was 12.1±1.8 for the wild type and 11.6±2.2 forsec22-3(n=6). Germination rates were identical on soil (86%±2% in wild type and 88%±2% insec22-3) as well as in hydroponic culture (100% in wild type and 95%±2% insec22-3). Data are presented as means±s.d.;n≥20. (b) The mutant did not reveal obvious developmental defects in comparison with wild type; in particular, flower development was not altered. Size bars: upper panel 0.5 cm; lower panel 2 cm. Full size image Figure 6: Growth of A. thaliana wild type and sec22-3 . ( a ) Plant development was quantified by measuring biomass (fresh weight) of aerial parts at the indicated time points ( n ≥15). Fresh weight to dry weight ratio was 12.1±1.8 for the wild type and 11.6±2.2 for sec22-3 ( n =6). Germination rates were identical on soil (86%±2% in wild type and 88%±2% in sec22-3 ) as well as in hydroponic culture (100% in wild type and 95%±2% in sec22-3 ). Data are presented as means±s.d. ; n ≥20. ( b ) The mutant did not reveal obvious developmental defects in comparison with wild type; in particular, flower development was not altered. Size bars: upper panel 0.5 cm; lower panel 2 cm. 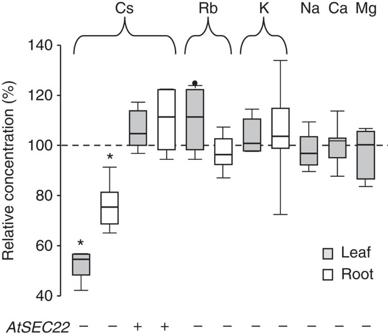Figure 7: Cation phenotype of theA. thalianainsertion mutantsec22-3. Cs+and Rb+accumulation in leaves and roots of 20-day-old wild-type andsec22-3plants were analysed in tracer uptake experiments; amounts are related to fresh weight. K+, Na+, Ca2+and Mg2+contents were measured by atomic emission spectroscopy and referred to dry weight. The fresh weight to dry weight ratio was not different between wild type andsec22-3(Fig. 6). Hundred percent correspond to 107±8.2 nmol Cs+g−1shoot (rosette); 43±6.6 nmol Cs+g−1root; 158±7.7 nmol Rb+g−1shoot; 53±7.4 nmol Rb+g−1root; 1.3±0.4 mmol K+g−1shoot; 0.62±0.08 mmol K+g−1root; 0.2±0.003 mmol Na+g−1shoot; 0.15±0.01 mmol Ca2+g−1shoot; and 0.3±0.01 mmol Mg2+g−1shoot (n≥5, each replicate consisting of at least six plants). Box plots with upper/lower quartiles, minimal and maximal values (antennas), and one outlier (black dot) are shown; asterisks indicate significant differences from wild type (P≤0.001,t-test). The expression ofAtSEC22is indicated as + (complemented line) or − (mutant). Full size image Figure 7: Cation phenotype of the A. thaliana insertion mutant sec22-3 . Cs + and Rb + accumulation in leaves and roots of 20-day-old wild-type and sec22-3 plants were analysed in tracer uptake experiments; amounts are related to fresh weight. K + , Na + , Ca 2+ and Mg 2+ contents were measured by atomic emission spectroscopy and referred to dry weight. The fresh weight to dry weight ratio was not different between wild type and sec22-3 ( Fig. 6 ). Hundred percent correspond to 107±8.2 nmol Cs + g −1 shoot (rosette); 43±6.6 nmol Cs + g −1 root; 158±7.7 nmol Rb + g −1 shoot; 53±7.4 nmol Rb + g −1 root; 1.3±0.4 mmol K + g −1 shoot; 0.62±0.08 mmol K + g −1 root; 0.2±0.003 mmol Na + g −1 shoot; 0.15±0.01 mmol Ca 2+ g −1 shoot; and 0.3±0.01 mmol Mg 2+ g −1 shoot ( n ≥5, each replicate consisting of at least six plants). Box plots with upper/lower quartiles, minimal and maximal values (antennas), and one outlier (black dot) are shown; asterisks indicate significant differences from wild type ( P ≤0.001, t -test). The expression of AtSEC22 is indicated as + (complemented line) or − (mutant). Full size image The chemical similarity of the non-essential alkali cation Cs + with the essential K + is a major obstacle for genetic attempts to manipulate radiocaesium accumulation and to prevent it from entry into the food chain [5] , [6] , [9] . In this study, however, we demonstrate that specific discrimination against Cs + is possible in the yeast s ec22Δ mutant, while other cations including K + are retained at wild-type levels. Surprisingly, the loss of the orthologous A. thaliana SEC22 expression in vegetative tissues also specifically lowered Cs + concentrations in plants ( Figs 1 and 7 ). Mathematical modelling and biochemical characterization of the yeast mutant reveals that Cs + sequestration to the vacuole is strongly compromised. The specific effect of the loss of Sec22p on Cs + uptake is further supported by the different uptake time courses of mutants constricting plasma membrane cation influx or efflux. In addition, these experiments under high-affinity conditions clearly confirm the suspected role of Trk1p and Trk2p in Cs + influx across the plasma membrane [8] , [24] and, conversely, the impact of Ena1-4p-driven cation transport in Cs + extrusion from the cells. The Cs + uptake time courses show an interesting biphasic behaviour with an initial plateau for both wild-type and sec22Δ mutant cells before further accumulation proceeds. This observation suggests a threshold leading to the onset of further Cs + sequestration to the vacuole. A similar behaviour has been observed for trk1Δ , although the second phase has been delayed, whereas in ena1-4Δ the initial phase is apparently lacking. Both findings could be in agreement with a lagging Cs + influx in trk1Δ or a more rapid Cs + accumulation in ena1-4Δ . Discrimination against Cs + at the vacuole in sec22Δ mutants is specific with respect to the essential cation K + . The total K + concentration and the Rb + compartmentalization have not been different from the wild type, which indicates unchanged vacuolar K + levels. Vacuolar K + concentration was estimated to be about 440 mM for both wild-type and sec22Δ cells based on (i) the relative volumes of the compartments, (ii) the measured total concentration of K + in whole cells ( Fig. 1 ) and (iii) the assumption of a vacuolar partitioning of K + analogous to Rb + ( Fig. 2e ). The corresponding cytosolic K + concentration is ~63 mM. Furthermore, the specificity of Cs + sequestration to the vacuole is supported by the consideration that even minor changes in the vacuolar K + concentration of sec22Δ would substantially decrease the total K + level (which has not been observed) provided that the cytosolic K + homeostasis must be preserved to retain a wild-type-like growth and viability in the sec22Δ mutant [26] . In contrast to our findings, Fell et al. [27] had also suggested an effect on K + homeostasis in sec22Δ based on an attenuated Rb + accumulation in the early phase of an uptake experiment in nutrient-deficient medium. An altered K + homeostasis was shown to affect the sensitivity to cationic drugs [28] and thus could be also related to the Cs + phenotype of sec22Δ . However, in contrast to nutrient-deficient medium, the early uptake time course of Rb + is identical for wild type and sec22Δ in YPD-rich medium ( Supplementary Fig. S6 ) and the steady-state Rb + and K + concentrations are not affected either (see above). Sec22p/SEC22 seems to be essential for the uptake and sequestration of Cs + in the wild type, as its loss of function leads to specifically reduced Cs + uptake in yeast and Arabidopsis . The SNARE Sec22p has been implicated in diverse aspects of protein targeting and autophagy (see the first section of text). Sec22p’s classical role as a v-SNARE is in the early anterograde vesicle transport [29] . Results of this work suggest a further link to vacuoles. A direct involvement of the ER-/Golgi-resident Sec22p to vacuolar membranes has been indicated by the fusion of proteoliposomes carrying the R-SNARE Sec22p and vacuolar Qabc-SNAREs. Although the R-SNARE contributes little to fusion specificity and the in vivo relevance has not been studied, this work demonstrates the biophysical ability of Sec22p to interact with vacuolar membranes [30] . Another link to vacuolar functions is provided by the co-responsiveness of Sec22 and Vma22 in the yeast transcriptome [31] . The ER-resident Vma22p is required for assembly of the V-ATPase, which acidifies the vacuolar lumen [32] . Diminished V-ATPase activity results in increased pH sensitivity and in repressed cation uptake into the vacuole [33] . However, sec22Δ exhibits only weak pH sensitivity in comparison with vma22Δ and the V-ATPase subunit mutant vma2Δ ( Fig. 3e ) [32] , [34] . This observation suggests that the sec22Δ Cs + phenotype is not owing to a disturbance of vacuolar pH, which is also in agreement with the unchanged K + and Rb + homeostasis in the SNARE mutant ( Fig. 1 ). Therefore, Sec22p apparently has a more specialized, non-redundant role affecting the specificity of Cs + deposition to vacuole. Although the detailed molecular mechanism remains obscure, with regard to the known functions of Sec22p and its potential additional link to the vacuole, it may be involved in targeting transporters or transport specificity-modulating proteins to alter the efficacy of cation sequestration to the vacuole. Potential targets to be altered at the tonoplast are the H + /cation exchange proteins Vnx1p and Nhx1p [35] , [36] , [37] . In addition, the loss of sec22Δ could lead to mistargeting of such proteins. Recently, the partial mistargeting of plasma membrane Trk1p to a yet undetermined intracellular compartment in the sec22Δ mutant background has been reported [27] . The successful transfer of the Cs + -discriminative phenotype from the unicellular yeast model to a higher plant has implications for possible strategies towards breeding ‘safer crops’. Although the Arabidopsis SEC22 is essential for proliferation [18] , this work shows that its specific loss of function in vegetative tissue allowed for wild-type-like growth and development, yet reducing Cs + accumulation ( Figs 6 and 7 ). Therefore, an organ-specific suppression of SEC22 could reduce the entry of radiocaesium into the food chain, which could be also employed in conjunction with other approaches, such as manipulation of K + -transporter specificity or agricultural measures like K + -rich fertilization [5] . The conservation of SEC22 homologues in crop species supports such a strategy. Chemicals All chemicals were purchased at the highest available grade from Sigma (Germany), Merck (Germany), VWR (Germany) or Serva (Germany). Radiochemicals were obtained from AEA Technology (Germany), GE Healthcare (Germany) or Hartmann Analytics (Germany). Yeast strains and growth conditions Mutant strains sec22Δ, vps35Δ, apl4Δ and aps3Δ are isogenic to BY4741 (MATa; his2Δ1; leu2Δ0; met15Δ0; ura3Δ0 ) and were obtained from EUROSCARF (Institute of Molecular Biosciences, University of Frankfurt). trk1Δ (PLY234) , trk2Δ (PLY236) and trk1Δtrk2Δ (PLY240) are isogenic to PLY232 (MATa; his3Δ200 leu2-3,112 trp1Δ901 ura3-52 suc2Δ9 ) (ref. 24 ). ena1-4Δ (G-19) is isogenic to W303.1 (ref. 23 ). Yeast transformation was performed by addition of 500 ng plasmid DNA to 75 μl of exponentially grown yeast cells permeabilized by lithium acetate [38] . A 3 kb genomic fragment encompassing the yeast Sec22 gene was amplified with primers SEC22coXmaIfw and SEC22coHindIIIrv ( Supplementary Table S5 ) and inserted into the plasmid Yep352 after restriction with Xma I and Hin dIII for complementation of sec22Δ (ref. 39 ). For complementation of yeast sec22Δ with Arabidopsis SEC22 ( At1g11890 ), the open reading frame was amplified using the oligonucleotides SEC22fwClaI and SEC22revNotI ( Supplementary Table S5 ) and cloned into the vector pCM189 [40] after restriction with Cla I and Not I, which allowed doxycyclin-repressible expression. Yeast cells were grown on YPD medium, pH 6.0 at 30 °C, if not noted otherwise [41] . The mutants trk1Δ , trk2Δ and trk1Δ trk2Δ , as well as their corresponding wild-type strains, were grown in YPD supplemented with additional 100 mM KCl. Yeast caesium and rubidium uptake assays Cs + accumulation assays in 96-well MultiScreen HTS plates (Millipore, Germany) were performed using 1 × 10 7 cells per well in 200 μl. Cells were incubated in YPD-rich medium, which was supplied with 50 μM 5-fluorouracil (5-FU) 4 h before the start of tracer incubation. This caused growth and cell division arrest without affecting the viability of yeast, in accordance with literature [42] . After washing with H 2 O, cells were resuspended in 100 μl YPD plus 50 μM 5-FU. After 1 h regeneration, an equal amount of YPD supplemented with 50 μM 5-FU and 100 μM CsCl containing 4 kBq ml −1 134 Cs was added. The plates were incubated at 30 °C on a shaker at 100 r.p.m. Assays were stopped by washing the cells twice before γ-spectrometric analysis. This experimental setup allowed quasi-constant uptake conditions, as the 50 μM external Cs + was at most depleted to 44 μM. A similar approach was followed for the determination of the Rb + content after 18 h using 50 μM RbCl containing 10 kBq ml −1 86 Rb as a radioactive tracer. In addition, an initial phase of Rb + accumulation in wild-type BY4741 and sec22Δ were performed in nutrient-limited conditions (50 mM HEPES Tris, pH 7.0 supplied with 2% glucose) without the addition of 5-FU in comparison with rich medium. For an efflux experiment, yeast cells incubated in 50 μM 134 Cs tracer-containing YPD containing 50 μM of 5-FU were harvested after 18 h and washed twice with tracer-free medium. Cells were incubated in tracer-free medium containing 50 μM CsCl at 30 °C and analysed at defined time points as cells above. Sensitivity analysis of yeast strains For cation toxicity tests, yeast cells were replica plated on YPD plates supplemented with different concentrations of NaCl, KCl and CsCl. For testing pH sensitivity, a dilution series of overnight cultures (OD 600 =0.8–1.0) was grown on selective YPD plates with different pH, adjusted with 20 mM MES-NaOH (pH 5.5 and 6.5) or 20 mM HEPES-NaOH (pH 7.5 and 8.0). Isolation of intact vacuoles to analyse Cs + partitioning Vacuoles were isolated by a stepwise Ficoll density gradient from spheroplasts obtained from 1 l tracer-laden cells (OD 600 =0.8) (refs 41 , 43 , 44 ). Yeast cells had been incubated at 30 °C for 18 h in YPD containing 50 μM 5-FU with 50 μM CsCl or RbCl, labelled with 50 kBq l −1 134 Cs or 500 kBq l −1 86 Rb, respectively. After enzymatic cell wall digestion, all steps were performed at 0 °C to reduce a potential loss of Cs + . Cells were osmotically lysed by Dounce homogenization in 10 mM Tris-MES, pH 6.9, 12% Ficoll, 0.1 mM MgCl 2 and 500 U ml −1 protease inhibitor cocktail (Sigma, Germany). After ultracentrifugation (30 min, 50,000 g ), the pellet was retained as fraction 1. The floating material was isolated and overlaid with 8 and 4% Ficoll for another centrifugation (45 min, 50,000 g ). The pellet (fraction 2) and the floating vacuolar fraction (fraction 3) were collected. α-mannosidase activity in 134 Cs tracer-laden cell lysates was determined in 2 ml aliquots and the lysates were diluted to match the enzyme activity of the isolated vacuoles in a 6 ml volume. Enzymatic tests for yeast cell fractionation Marker enzyme assays were used to characterize the fractions obtained by density gradient fractionation ( Supplementary Fig. S4 ). All fractions were adjusted to the same volume (500 μl) before aliquots were analysed. Spheroplasts were used as whole-cell reference. All activities refer to equivalent portions of the individual fractions. Vanadate-sensitive plasma membrane ATPase activity was quantified by the vanadate-sensitive release of phosphate from ATP in the presence of 5 mM sodium azide [45] , [46] . The peroxisomal marker catalase A was assayed by the titanium oxysulfate method [47] , [48] . NADPH cytochrome c reductase was used as an ER marker based on the reduction of cytochrome c in the presence of NADPH and rotenone [48] . The activity of α-1,6-mannosyltransferase was assayed as a Golgi marker using GDP-[ 14 C]-mannose and α-1,6-mannobiose as substrates [49] , [50] . The mitochondrial marker succinate dehydrogenase was assayed by quantifying reduced p -iodonitrotetrazolium violet [48] , [51] . Finally, carboxypeptidase Y and a- D -mannosidase were employed as markers for the vacuolar lumen and membrane, respectively [28] , [52] , [53] . Carboxypeptidase Y activity was based on the release of leucine from N-CBZ- L -Phe- L -Leu. Activity of α- D -mannosidase was measured using p -nitrophenyl-α- D -mannopyranoside as a substrate. Plant lines and growth conditions Wild-type control plants were A. thaliana accession Col-0. The T-DNA insertion line SALK_042619 ( sec22-3 ) was obtained from Nottingham Arabidopsis Stock Centre [54] , [55] and verified by DNA sequencing. Homozygous insertion lines were selected by PCR ( Supplementary Table S5 ) and characterized by RT–PCR ( Fig. 4b and Supplementary Table S4 ). Plants were grown either in hydroponics after seed surface sterilization [14] or on a non-fertilized, irrigated soil-sand substrate after stratification for 2 days with 16 h light (75 μmol m −2 s −1 ) at 21 to 23 °C. Complementation of A. thaliana sec22-3 The Arabidopsis SEC22 gene ( At1g11890 ) was reassembled from fragments obtained by PCR with primer combinations (I) PromSecfwXmaI ,+ PromSecrevClaI , (II) SEC22fwClaI + SEC22revXhoI and (III) TermSecfwXhoI + TermSecrevPstI ( Supplementary Table S5 ) and subsequent restriction digestion ( Xma I, Cla I, Xho I or Pst I). These fragments were ligated into vector pBGW [55] , [56] cut by Xma I and Pst I. The correct sequence was verified by DNA sequencing. sec22-3 plants were transformed using the floral dip method with Agrobacterium tumefaciens pGV301/pMP90 containing the pBGW derivative [57] . A homozygous line carrying a single insertion was used for further analysis. γ-Spectrometric analysis of 134 Cs and 86 Rb Yeast cells were dissolved in 3 ml 3 M HNO 3 before γ-spectrometric analysis with 60 min counting in a Wallac WIZARD 1480 (Perkin Elmer, Germany) based on the spectral peaks for 134 Cs (605 and 796 keV) and 86 Rb (1077, keV). Yeast vacuolar fractions were analysed in 6 ml of the isolated fraction. For Arabidopsis samples, at least seven 20-day-old plants from hydroponic cultures supplemented with 5 μM CsCl containing 12 kBq l −1 134 Cs or 5 μM RbCl with 24 kBq l −1 86 Rb were pooled per replicate [14] . The aerial part (rosette including stem) was separated from the root below the hypocotyl. The material was washed once with water, dried briefly on tissue paper, resuspended in 3 ml H 2 O and analysed. Determination of non-labelled cation concentrations Yeast cultures were shaken (30 °C; 100 r.p.m.) for 18 h in 50 ml YPD containing 50 μM 5-FU. Cells (OD 600 ≈0.8) were collected on 45 μm filters and dissolved in 3 ml of 30% HNO 3 at 60 °C overnight. After a threefold dilution with H 2 O, 5 ml was analysed using inductively coupled plasma atomic emission spectrometry (Optima 7300, Perkin Elmer, Germany) equipped with a seaspray nebulizer fitting to a cyclon spray chamber (AHF Analysentechnik, Germany). The following elemental emission lines were measured: Ca 2+ : 317.933 nm; K + : 766.490 nm; Mg 2+ : 279.077 nm; and Na + : 589.592 nm. Concentrations were determined by external calibration. Arabidopsis roots and leaves from at least eight rosettes or root systems were pooled per sample. Cations were determined by atomic emission spectrometry as above from 2 mg freeze-dried roots or rosette leaves. Microscopy Microscopic analyses were performed with an Olympus BX61 equipped with software Cell*P (Olympus, Europe). Yeast cells and vacuoles were counted in a Neubauer-type haemocytometer. Cellular and vacuolar volumes were determined after staining cells (OD 600 <1.0) with 15 μM SynaptoRed C2 (=FM4-64) (Biotium, CA, USA; 525 nm excitation, 647 nm emission), which was also used as viability indicator [58] . The cellular (35 fl) and vacuolar (9 fl) volumes for wild type under our experimental conditions are in accordance with literature [59] . How to cite this article: Dräxl, S. et al. Caesium accumulation in yeast and plants is selectively repressed by loss of the SNARE Sec22p/SEC22. Nat. Commun. 4:2092 doi: 10.1038/ncomms3092 (2013).